Available data do not rule out Ctenophora as the sister group to all other Metazoa 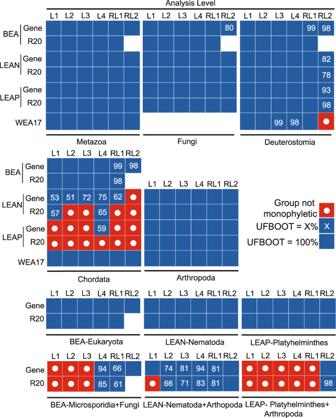Fig. 1: Inference of benchmark relationships following phylogenetic approaches used by Redmond and McLysaght1with partitioning by gene and partitioning using 20% relaxed clustering. Dataset and analysis level abbreviations follow Redmond and McLysaght1. “Gene” and “R20” reflect whether the analysis was partitioned by gene or by using 20% relaxed clustering. L1, L2, L3, and L4 are non-recoded analyses with increasing use of site-heterogenous models (see methods of RM). RL1 is recoded analyses without site-heterogeneous models and RL2 is recoded analyses with site heterogeneous models. Solid blue boxes indicate 100% ultrafast bootstrap (UFBOOT) support for the relationship labelled under each set of boxes (e.g., “Metazoa”, “Fungi”). Numbers represent ultrafast bootstrap support less than 100%. Red boxes with dots indicate that a relationship was not recovered. Analysis RL2 for BEA is not reported as IQTREE 1.6.12 tree inference failed because of an error, likely resulting from overparameterization. Maximum likelihood trees were inferred with non-recoded and SR [3] recoded datasets BEA, LEAP, and LEAN from RM [1] . Following RM [1] , six analyses were done on each dataset (i.e., L1, L2, L3, L4, RL1, RL2) to test for the influence of including site-heterogenous models in analyses. Best-fit partitions and substitution models were inferred with ModelFinder [12] , as implemented in IQ-TREE 1.6.12 [2] , with 20% relaxed clustering; branch lengths were linked and each partition was allowed to have its own evolutionary rate. For model testing, L1 analyses included only standard site homogeneous protein subtitution models (e.g., Dayhoff, JTT), L2 analyses included all models from L1 analyses and multi-matrix models (e.g., EX2, LG4M), L3 analyses included all models from L1 and L2 analyses plus multi-profile models with Poisson exchangeabilities (e.g., C10, C20), and L4 analyses included all models from L1, L2, and L3 analyses plus multi-profile models with non-Poisson exchangeabilities (e.g., JTT + C10, LG-C30). Model testing for RL1 analyses included site-homogeneous nucleotide (i.e., 4-state) models. Model testing for RL2 analyses included all models from RL1 analyses plus multi-profile site-heterogenous models with either Poisson or GTR exchangeabilities. All analyses included testing models with a parameter for rate heterogeneity. Following RM [1] , partition finding was done only on L1 analyses; model-testing for L2, L3, L4, RL1, and RL2 analyses was done with the best-fit partitions from L1 analyses on each dataset. Model testing, as described above, was consistent with what was done by RM on the same datasets but with IQ-TREE 1.6.12. Tree inference was done with IQ-TREE using best-fit paritions and models. Support was assessed with 1000 ultrafast boostrap replicates [13] . Reporting summary Further information on research design is available in the Nature Portfolio Reporting Summary linked to this article.